Carbon isotope records reveal precise timing of enhanced Southern Ocean upwelling during the last deglaciation The Southern Ocean plays a prominent role in the Earth’s climate and carbon cycle. Changes in the Southern Ocean circulation may have regulated the release of CO 2 to the atmosphere from a deep-ocean reservoir during the last deglaciation. However, the path and exact timing of this deglacial CO 2 release are still under debate. Here we present measurements of deglacial surface reservoir 14 C age changes in the eastern Pacific sector of the Southern Ocean, obtained by 14 C dating of tephra deposited over the marine and terrestrial regions. These results, along with records of foraminifera benthic–planktic 14 C age and δ 13 C difference, provide evidence for three periods of enhanced upwelling in the Southern Ocean during the last deglaciation, supporting the hypothesis that Southern Ocean upwelling contributed to the deglacial rise in atmospheric CO 2 . These independently dated marine records suggest synchronous changes in the Southern Ocean circulation and Antarctic climate during the last deglaciation. Knowledge of marine surface reservoir radiocarbon ages ( R surf , that is, the difference between the 14 C age of the sea surface and that of the atmosphere) allows the accurate correlation of continental, cryospheric and marine palaeoclimate records. Accurate comparison of palaeoclimate records is essential in order to understand the timing, causality and mechanisms of past climate changes. Besides enhancing the accuracy of age models, R surf reconstructions also provide clues about past changes in ocean circulation patterns [1] , [2] , [3] , some of which have been linked to the rise in atmospheric CO 2 over the last deglaciation [4] , [5] , [6] , [7] , [8] . In this respect, the Southern Ocean (SO), which connects the deep ocean with surface waters and the atmosphere, plays a major role in global ocean circulation and the carbon cycle [4] , [9] . It has been proposed that SO upwelling, the intensity of which depends partly on changes in the strength and position of Southern Hemisphere westerly winds, could be the primary route for ocean CO 2 degassing during the last deglaciation [4] , [5] , [6] , [7] , [8] , [10] , [11] , [12] , [13] . This so-called SO upwelling hypothesis remains a controversial issue. On one hand, records from intermediate depths in the South East Pacific (SEP) have shown a reduction in Antarctic Intermediate Water (AAIW) oxygen concentration during the deglacial warming period, which may be linked with an upwelling of low oxygen waters at the SO divergence, which are transported northward via AAIW [14] . On the other hand, 14 C records from the South Pacific do not indicate any deglacial 14 C depletion at intermediate depths off Chile and New Zealand [11] , [13] , which does not support the SO upwelling hypothesis. Part of the controversy may arise from potentially biased chronologies in marine sediment cores for which it is difficult to derive robust estimates of R surf . Only one study has provided independent R surf in the southwest Pacific Ocean [3] during the glacial period; however, there are no estimates for the SO during the deglaciation. Deep-sea coral records can provide robust chronologies for deep waters because of the direct comparison between U/Th and 14 C ages; however, they do not ensure a simultaneous climatic record for bottom and surface waters [15] . The precise dating of SO ventilation records is, however, crucial in linking CO 2 outgassing events, and their timing, to changes in atmospheric CO 2 concentrations recorded in ice cores. Here we present the first deglacial Pacific SO record of R surf based on the occurrence of tephra layers independently dated in the ocean and on land. The well-dated marine tephra used in this study is identified in the sediment core MD07-3088 collected off the southern Chilean margin (North Patagonia) at a depth of 1,536 m ( Fig. 1 ). The core is located within the Antarctic Circumpolar Current (ACC) under the direct influence of the northward Ekman transport of Sub-Antarctic Surface Waters (SSW) [16] ( Fig. 1a,b ). Today, the core depth is bathed by the upper layers of the nutrient-rich, oxygen-poor Pacific Central Waters at the boundary with the northward-flowing oxygen-rich AAIW. Thus, this core is well located to monitor the past SO upwelling history. We show that R surf at this location is larger during the deglaciation than during the Holocene and that periods of increased R surf are coeval with periods of increased SO vertical mixing. These precisely dated palaeoceanographic records indicate a strong correlation between SO upwelling events and the deglacial atmospheric CO 2 rise, providing strong support for the SO upwelling hypothesis. The R surf reconstructions also help to reveal a deglacial ageing of AAIW that is consistent with its reduction in oxygen concentration [14] , indicating that deglacial CO 2 excess was spread, at least partly, via an AAIW pathway. 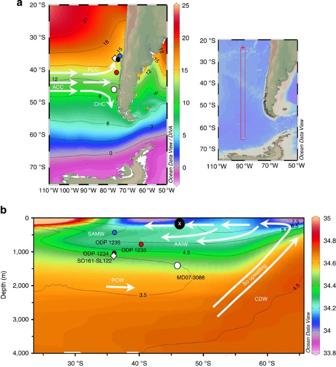Figure 1: Study area and core locations. (a) Map of the mean annual SST (°C) using the Ocean Data View (ODV) software56and geographical locations of cores MD07-3088 (46 °S, 75 °W, 1,536 m; white circle), ODP 1233 (41 °S, 74 W, 838 m; solid red circles14), ODP 1234 (36 °S, 73 °W, 1,015 m; solid black circles14), ODP 1235 (36 °S, 73 °W, 489 m; solid blue circles14), and SO161-SL122 (36 °S, 73 °W, 1,000 m; white diamond11). ACC: Antarctic Circumpolar Current. PCC: Peru–Chile Current. CHC: Cape Horn Current. The inset on the map corresponds to the transect for the latitude-depth section presented inb. (b) Salinity (psu, coloured shading) and oxygen (ml l−1, thin black contours) depth-latitude section. SAMW: Sub-Antarctic Mode Waters. AAIW: Antarctic Intermediate Water. PCW: Pacific Central Water. CDW: Circumpolar Deep Water. The filled circle with cross indicates the flow of SSW. Core location is indicatively plotted following the inset ofFig. 1aat the same collected depth and latitude but at different longitude. Figure 1: Study area and core locations. ( a ) Map of the mean annual SST (°C) using the Ocean Data View (ODV) software [56] and geographical locations of cores MD07-3088 (46 °S, 75 °W, 1,536 m; white circle), ODP 1233 (41 °S, 74 W, 838 m; solid red circles [14] ), ODP 1234 (36 °S, 73 °W, 1,015 m; solid black circles [14] ), ODP 1235 (36 °S, 73 °W, 489 m; solid blue circles [14] ), and SO161-SL122 (36 °S, 73 °W, 1,000 m; white diamond [11] ). ACC: Antarctic Circumpolar Current. PCC: Peru–Chile Current. CHC: Cape Horn Current. The inset on the map corresponds to the transect for the latitude-depth section presented in b . ( b ) Salinity (psu, coloured shading) and oxygen (ml l −1 , thin black contours) depth-latitude section. SAMW: Sub-Antarctic Mode Waters. AAIW: Antarctic Intermediate Water. PCW: Pacific Central Water. CDW: Circumpolar Deep Water. The filled circle with cross indicates the flow of SSW. Core location is indicatively plotted following the inset of Fig. 1a at the same collected depth and latitude but at different longitude. Full size image Climatic record in core MD07-3088 Climatic conditions of surface waters at core MD07-3088 are recorded in the stable oxygen isotopes (δ 18 O) of planktonic foraminifera Globigerina bulloides ( Fig. 2a ) and the summer sea–surface temperature (SST), obtained by planktonic foraminifera assemblages and the Modern Analogue Technique ( Fig. 2b ). The δ 18 O and SST records show variations characteristic of the last glacial/interglacial transition and the Holocene, with two warming phases (W1 and W2) separated by a reversal to colder conditions (Oceanic Cold Reversal or OCR) ( Fig. 2 ). Both the δ 18 O and SST records display short-term variability within each climatic phase, potentially indicating abrupt hydrographic changes. 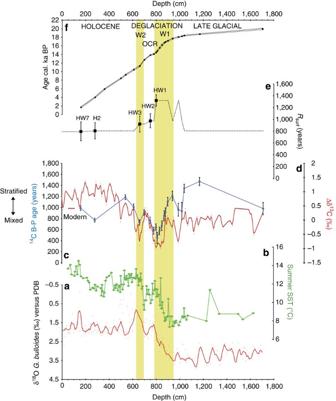Figure 2: Records and age control of core MD07-3088. (a) δ18O (per mil versus PDB) ofG. bulloides. Smoothed curve using a three-point average (thick red line). (b) Summer Sea Surface Temperature (°C) using Modern Analogue Technique. (c)14C age difference between paired benthic and planktic foraminifera (14C B-P; filled squares). The error bars represent combined error at 1. Red dash: modern B-P14C age24. Double-ended arrow indicates stratified (higher14C B-P and Δδ13C values) versus mixed (lower14C B-P and Δδ13C values) water mass. (d) Δδ13C=δ13CG. bulloides—δ13CC. wuellerstörfii(red dots). Smoothed curve using a three-point average (thick red line). (e)Rsurfage (squares) and assumedRsurf(dotted line) in core MD07-3088. HW7, H2, HW3, HW2, HW1: terrestrial tephra from the Hudson volcano (Supplementary Table S1). The error bars represent combined error at 1σ. (f) Calibrated14C ages (ka BP) versus depth with 1σ uncertainties. OCR: Ocean Cold Reversal. W1 and W2 (yellow shading): the two Southern Ocean warming phases of the last deglaciation. Figure 2: Records and age control of core MD07-3088. ( a ) δ 18 O (per mil versus PDB) of G. bulloides . Smoothed curve using a three-point average (thick red line). ( b ) Summer Sea Surface Temperature (°C) using Modern Analogue Technique. ( c ) 14 C age difference between paired benthic and planktic foraminifera ( 14 C B-P; filled squares). The error bars represent combined error at 1. Red dash: modern B-P 14 C age [24] . Double-ended arrow indicates stratified (higher 14 C B-P and Δδ 13 C values) versus mixed (lower 14 C B-P and Δδ 13 C values) water mass. ( d ) Δδ 13 C=δ 13 C G. bulloides —δ 13 C C. wuellerstörfii (red dots). Smoothed curve using a three-point average (thick red line). ( e ) R surf age (squares) and assumed R surf (dotted line) in core MD07-3088. HW7, H2, HW3, HW2, HW1: terrestrial tephra from the Hudson volcano ( Supplementary Table S1 ). The error bars represent combined error at 1σ. ( f ) Calibrated 14 C ages (ka BP) versus depth with 1σ uncertainties. OCR: Ocean Cold Reversal. W1 and W2 (yellow shading): the two Southern Ocean warming phases of the last deglaciation. Full size image Radiocarbon ages and stable carbon isotopes R surf estimates are based on detailed geochemical analyses and 14 C dating of both terrestrial and marine tephra deposits ( Supplementary Table S1 ; Fig. 2e ). Over the last deglaciation, five tephra showed that R surf was at 1,320±95 years at the end of the first phase of deglacial warming (W1 on Fig. 2 , HW1 tephra). R surf decreased to 975±120 years during the OCR (HW2 tephra), to 920±135 years during the second warming phase (W2 on Fig. 2 , HW3 tephra) and to 800 years during the Holocene (H2 and HW7 tephra; Fig. 2e ). Today, pre-bomb R surf is poorly documented in the SEP, except for one single available date at 530±40 years from the southern Chilean fjords (51 °S, 72 °E (ref. 17 )). This fjord site is not likely to be representative of open ocean conditions, as it is largely affected by local conditions such as melt-water supply [18] . Our results indicate that the youngest R surf estimates at ca . 800 years, obtained from core MD07-3088 during the upper Holocene, are similar to those obtained during the Middle Holocene and are in agreement with other studies carried out along the SEP margin, as well in the SO, which have revealed no changes in regional R surf during this period [19] , [20] , [21] , [22] . As a consequence, middle to upper Holocene R surf estimate at ca . 800 years along the Southern Chilean margin at 46 °S can be regarded as the most plausible for the pre-bomb period. We assume that the large R surf changes during the deglacial period in core MD07-3088 cannot be because of contamination by old carbon carried by the Aisén and northern Patagonian tributary rivers, as the main geological units of the Coastal Range and Cordillera are composed primarily of pre-Jurassic metamorphic basement, ophiolite, plutonic rocks and volcanic material [23] . This assumption is supported by the δ 18 O and δ 13 C records of the planktic foraminifera G. bulloides from MD07-3088 and a farther offshore core, MD07-3119 (46°05 S, 76°06 W, 2,520 m), recovered at the same latitude ( Supplementary Fig. S1 ). The results show similar δ 18 O and δ 13 C oscillations during the deglaciation and early Holocene, clearly indicating that the core MD07-3088 signals are representative of the open ocean and are not influenced by local coastal effects. R surf changes can result from changes in the atmospheric 14 C activity or from variations in the exchange of surface waters with the atmosphere and underlying 14 C-depleted waters. Variability in vertical mixing (stratification) is effectively recorded in differences between the carbon isotope composition of benthic and planktonic foraminifera (B-P 14 C age and Δδ 13 C). We evaluate the influence of changing atmospheric 14 C activity on B-P ages using an ocean circulation model (see Methods). B-P age differences were ~1,400 14 C years during the Late Glacial, ~400 years higher than modern values (modern B-P is ~1,000 years [24] ), suggesting more stratification and poorly ventilated deep-water masses in the SEP region ( Fig. 2c ; Supplementary Table S2 ). The late glacial–interglacial transition is marked by three periods of low values for B-P age, coeval with three periods of low Δδ 13 C values ( Fig. 2d ). The end of the first short decrease in the B-P age and Δδ 13 C marks the onset of the deglaciation, followed by two longer periods of low values. During the first warming episode W1, the B-P age reaches its minimum value of 450 years. Then, B-P age and Δδ 13 C increase during the OCR, prior to a third period of low values during the second warming W2 ( Fig. 2c,d ). Thus, the oldest R surf , at 1,320±95 years, which occurred during the minima of the B-P age within the episode W1, could originate from enhanced upwelling of 14 C-depleted deep waters. Age model and mechanisms for R surf changes To establish the chronology of the core, we used 24 14 C ages on planktic foraminifera corrected with the R surf age determined from the tephra layers ( Fig. 2f ). Then, the R surf -corrected planktic 14 C dates were calibrated using the OxCal software [25] based on the IntCal09 (ref. 26 ) calibration curve. We also present most of the results using the IntCal04 (ref. 27 ) calibration curve as it critically deviates from IntCal09 during 17.5 to 15ka BP, in line with recent nonmarine data from speleothems [28] and varved lake sediments [29] . 14 C data and R surf estimates are reported in Supplementary Tables S1,S2 . Prior to the HW1 tephra, marine ash layers found in the core could not be correlated to dated terrestrial volcanic products [30] . To date, existing continental records west of the Andes do not extend beyond 15 ka because of the presence of a permanent icecap in the region [31] . Before 14.5 ka, we apply the basic assumption of using the highest R surf (1,320 years from the HW1 tephra) when the B-P age and Δδ 13 C decrease ( Fig. 2 ), and the lowest R surf (800 years from the H2 and HW7 tephra) for times when the B-P age and Δδ 13 C are relatively constant. This approach is based on the observation that the major R surf increase in core MD07-3088, which occurred during the last deglaciation, is contemporaneous with the maximum decrease in B-P age difference, suggesting mixing with 14 C-depleted deep waters. The B-P age difference during the last glaciation is noticeably higher than that during the deglacial period, indicating well-stratified water masses and the fact that glacial atmospheric Δ 14 C was higher. A well-stratified water mass could lead to a reduced R surf during the late glacial period. However, it might have been compensated for by the higher glacial atmospheric Δ 14 C and the reduced air–sea CO 2 flux because of lower p CO 2 . Therefore, we assume that R surf during the last glaciation did not differ significantly from that of the Holocene period. The inferred decrease in the B-P age and Δδ 13 C variations ( Fig. 3a,b ) originate either from enhanced vertical mixing in the SO (as for the HW1–HW2 period when R surf shows an opposite trend to the B-P age) or from rapid changes of the atmospheric δ 13 C compositions. In the atmosphere, two decreases have been observed in the δ 13 C signal [32] , [33] during the deglaciation ( Fig. 3d ); however, the amplitude of this atmospheric signal is only half that of the ocean surface δ 13 C that we have measured ( Fig. 3c ). Similarly, we checked that rapid decreases in atmospheric Δ 14 C ( Fig. 3g (refs 27 , 28 )) could not entirely explain the amplitude and timing of the decreases in the B-P age signal in core MD07-3088. The B-P age record, corrected for variations in atmospheric Δ 14 C, is shown in Fig. 3a with the raw B-P ages (see Methods). The similarity between the raw and the corrected B-P ages indicates that both carbon isotopic signals mainly reflect changes in SO upwelling. Furthermore, the largest and longest period of low Δδ 13 C and B-P age difference is associated with the highest R surf during the last deglaciation, emphasizing that SO upwelling provided a conduit for a 14 C-depleted deep-water mass to surface waters at that time ( Fig. 3a,b,f ). Conversely, during the OCR, a lowering of R surf to ~1,000 years mirrors the rise in Δδ 13 C and B-P age, indicating weaker SO upwelling. However, during W2, the next period characterized by both a lower Δδ 13 C and a slightly lower B-P age difference, the observed R surf changes vary little from their OCR value. Upwelled deep waters might have carried a much younger 14 C age during W2 than at the beginning of the deglaciation because of the first period of vertical convection in the SO and the resumption of deep-water formation in the North Atlantic after the Heinrich 1 event [34] . Another alternative is that the apparent B-P age decrease is because of variations in atmospheric Δ 14 C, as indicated by the B-P age data corrected for atmospheric Δ 14 C changes ( Fig. 3a ). One possible explanation for the apparent discrepancy in the R surf and δ 13 C records during W2 is that the production rate of 14 C in the atmosphere decreased during that time. If this were the case, an increase in upwelling might not be recorded as an increase in R surf . At the end of this third period of enhanced vertical mixing, R surf decreases towards its Holocene value, which is similar to the modern. 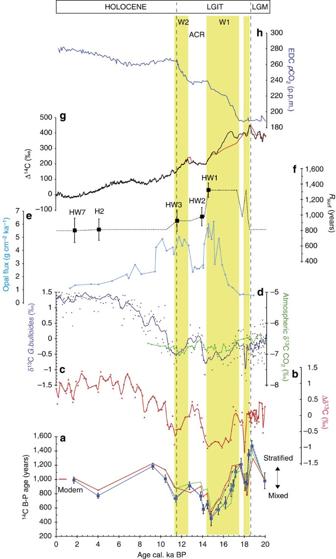Figure 3: Southern Ocean and atmospheric carbon cycle changes during the last deglaciation. (a) Paired benthic and planktic foraminifera radiocarbon age difference (14C B-P age; this study) using IntCal09 (thick blue line) and IntCal04 (dashed blue line) versus time. The error bars represent combined 1σ error in the radiocarbon dates. The B-P age difference corrected for Δ14C atmospheric changes (see Methods) is shown in red and green for IntCal04 and IntCal09, respectively. Double-ended arrow indicates stratified (higher B-P14C values) versus mixed (lower B-P14C values) water mass. Red dash: modern B-P14C age24. (b) Δδ13C in core MD07-3088; smoothed curve using a three-point average (thick red line). (c)G. bulloidesδ13C (this study); smoothed curve using a three-point average (thick purple line). (d) Ice core EDC δ13CO2measurements (green)32versus age scale from Lemieux-Dudonet al.36(e) Southern Ocean Opal flux, a proxy for upwelling south of the Antarctic polar front from core TN057-13-4PC (ref.5). (f)Rsurf(squares) and assumedRsurf(dotted line) in core MD07-3088. (g) Atmospheric14C activity (Δ14C), IntCal09 (black line), IntCal04 (red line)26,27. (h) Atmospheric CO2from ice-core EDC35. The vertical grey dashed lines indicate the approximate timing of Southern Hemisphere climatic events. LGIT: Last Glacial/Interglacial transition; ACR: Antarctic Cold Reversal; LGM: Last Glacial Maximum. Yellow shaded area: the three phases of Southern Ocean outgassing. W1 and W2: the two Southern Ocean warming phases of the last deglaciation. Figure 3: Southern Ocean and atmospheric carbon cycle changes during the last deglaciation. ( a ) Paired benthic and planktic foraminifera radiocarbon age difference ( 14 C B-P age; this study) using IntCal09 (thick blue line) and IntCal04 (dashed blue line) versus time. The error bars represent combined 1σ error in the radiocarbon dates. The B-P age difference corrected for Δ 14 C atmospheric changes (see Methods) is shown in red and green for IntCal04 and IntCal09, respectively. Double-ended arrow indicates stratified (higher B-P 14 C values) versus mixed (lower B-P 14 C values) water mass. Red dash: modern B-P 14 C age [24] . ( b ) Δδ 13 C in core MD07-3088; smoothed curve using a three-point average (thick red line). ( c ) G. bulloides δ 13 C (this study); smoothed curve using a three-point average (thick purple line). ( d ) Ice core EDC δ 13 CO 2 measurements (green) [32] versus age scale from Lemieux-Dudon et al . [36] ( e ) Southern Ocean Opal flux, a proxy for upwelling south of the Antarctic polar front from core TN057-13-4PC (ref. 5 ). ( f ) R surf (squares) and assumed R surf (dotted line) in core MD07-3088. ( g ) Atmospheric 14 C activity (Δ 14 C), IntCal09 (black line), IntCal04 (red line) [26] , [27] . ( h ) Atmospheric CO 2 from ice-core EDC [35] . The vertical grey dashed lines indicate the approximate timing of Southern Hemisphere climatic events. LGIT: Last Glacial/Interglacial transition; ACR: Antarctic Cold Reversal; LGM: Last Glacial Maximum. Yellow shaded area: the three phases of Southern Ocean outgassing. W1 and W2: the two Southern Ocean warming phases of the last deglaciation. Full size image The reconstructed age model for core MD07-3088 makes it possible to compare the EPICA Dome C (EDC) and SEP climatic records. Figure 3 illustrates the MD07-3088 records on a calendar age (cal.) scale, compared with the atmospheric δ 13 C [35] and isotopic compositions from the EDC ice core [32] , [36] and the record of atmospheric 14 C activity [26] , [27] . The planktic foraminifera δ 13 C record from core MD07-3088 shows a similar pattern to the δ 13 C of CO 2 inferred from the EDC ice core ( Fig. 3c,d (ref. 32 )). The excellent synchronicity of both records is particularly well documented for the rapid δ 13 C increase between 14.1 and 13.5 cal. ka BP in both our marine and the ice-core record. This event is chronologically very well constrained by two tephra, at 14.47±0.2 and 13.76±0.1 cal. ka BP, in our record and is synchronous with the δ 13 C rise of CO 2 according to the recent chronology of the EDC ice-core record [36] within the 1σ uncertainties. Here, for the first time, we are able to demonstrate a good synchronicity between climatic marine and cryospheric records in the Southern Hemisphere for a rapid event, displaying high temporal resolution (<150 years) and accurately dated boundaries. In general, the first order, and most of the second order, changes in the marine δ 13 C and δ 18 O and SSST records match well with the EDC δ 13 C and deuterium isotopic (δD) records during deglaciation ( Figs 3 , 4 ). Interestingly, for the SEP, the OCR cold spell is coeval with the Antarctic Cold Reversal event within the 1σ uncertainties ( Fig. 4a,b,d ). Moreover, in the SEP we do not see a delay as large as 800 years between the Antarctic Cold Reversal and OCR event as suggested for the South Indian Ocean [37] . These results are corroborated by the good match between the high-resolution Ti/K record and the EDC deuterium isotopic (δD) record ( Fig. 4c,d ). The Ti/K ratio has been used as a proxy to track past changes in the relative contribution of the terrigenous source derived from the volcanic area (high contents of Ti-rich minerals) of the Andean Cordillera versus that derived from the igneous rocks (high contents of K-rich minerals) of the Coastal Range [38] . These environmental changes have been attributed to climate fluctuations that occurred since the last glacial period in northern Patagonia and have been mainly related to precipitation and glacier behaviour [38] . 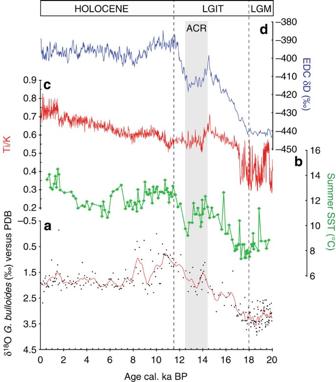Figure 4: Comparison of palaeoclimatic records from core MD07-3088 and EPICA DOME C. (a) Variations in δ18O (per mil versus PDB) ofG. bulloidesversus time. The thick red line corresponds to a smoothed curve using a three-point average. (b) Summer SST (°C) using the Modern Analogue Technique. (c) Ti/K ratio sedimentary record in core MD07-3088. (d) Ice-core deuterium (δD) record from EDC35based on the age scale of Lemieux-Dudonet al.36Note that the calendar age scale of the marine records (a-c) was determined in this study from marine radiocarbon data and is independent of the calendar age scale for the ice-core record (d). Vertical grey dashed lines indicate approximate timing of Southern Hemisphere climatic events. LGM=Last Glacial Maximum, LGIT=Last Glacial–Interglacial transition; ACR=Antarctic Cold Reversal. Figure 4: Comparison of palaeoclimatic records from core MD07-3088 and EPICA DOME C. ( a ) Variations in δ 18 O (per mil versus PDB) of G. bulloides versus time. The thick red line corresponds to a smoothed curve using a three-point average. ( b ) Summer SST (°C) using the Modern Analogue Technique. ( c ) Ti/K ratio sedimentary record in core MD07-3088. ( d ) Ice-core deuterium (δD) record from EDC [35] based on the age scale of Lemieux-Dudon et al . [36] Note that the calendar age scale of the marine records ( a - c ) was determined in this study from marine radiocarbon data and is independent of the calendar age scale for the ice-core record ( d ). Vertical grey dashed lines indicate approximate timing of Southern Hemisphere climatic events. LGM=Last Glacial Maximum, LGIT=Last Glacial–Interglacial transition; ACR=Antarctic Cold Reversal. Full size image The two steps in atmospheric CO 2 increase during the deglaciation [35] , from 17.4 to 14.4 ka and 12.5 to 11.5 ka, respectively [36] , are synchronous with the two latest periods of SO upwelling, indicated both by the B-P age and Δδ 13 C decrease in core MD07-3088 ( Fig. 3h , shaded areas W1 and W2). The precise timing of these core records supports the hypothesis that ocean CO 2 outgassing through SO upwelling is a major mechanism responsible for the deglacial atmospheric CO 2 rise [4] . The first period of SO upwelling, starting at ~18.4 cal. ka BP ( Fig. 3 , shaded area), occurs at the very beginning of the deglaciation as indicated by planktic foraminifera δ 18 O and by a recent composite record of Antarctic ice core temperatures [39] . This supports a coeval onset of Antarctic temperature and atmospheric CO 2 rise as suggested by recent studies on gas and ice-age difference of the ice cores [40] , [41] . The W1 and W2 upwelling periods identified in core MD07-3088 correspond to opal productivity events observed in the Atlantic and Pacific sectors of the SO (ref. 5 ) south of the polar front (core TN057-13-4PC; Fig. 3e ). However, the deglacial SO opal flux record does not register enhanced opal productivity during the first short-term period of SO upwelling recorded in core MD07-3088 at ~18.4 cal. ka BP. There are two possible explanations for this. First, it could be that the sedimentation rate in core TN057-13-4PC is not high enough to record so rapid an event. Second, it could be that the location of maximum opal production at the end of the last glacial maximum was shifted further north of the sub-antarctic zone and is therefore not recorded in this core [4] . The three periods of SO upwelling correspond to three rapid decreases in atmospheric Δ 14 C as indicated by the IntCal04 curve [27] ( Fig. 3g ). The major discrepancy between the IntCal09 (ref. 26 ) and IntCal04 (ref. 27 ) curves concerns the second deglacial event of SO upwelling. For this second event to be synchronous with the timing of the Δ 14 C decrease in IntCal09 (~16.35 cal. ka BP), the R surf should rise to up to 2,160±100 years. However, with such an increase in R surf , the second SO upwelling event would no longer be synchronous with the rapid CO 2 increase starting around 17.4 cal. ka BP ( Fig. 3g ). Moreover, the recently published complete terrestrial 14 C record for the 11.2–52.8 cal. ka BP interval [29] is more in agreement with the IntCal04 than the IntCal09 record. The inferred R surf changes outlined here enable us to reconcile several SEP marine palaeoceanographic studies at the regional scale and to clarify part of the controversy regarding the ventilation age history of AAIW. A recent compilation of the B-P 14 C age difference between paired benthic and planktic foraminifera from the central Chile margin ( Fig. 1 ; SO161-SL22; 36 °S, 73 °W; 1,000 m water depth; ref. 11 ) shows similar overall late Glacial to Holocene ventilation variations when compared with the MD07-3088 B-P record ( Fig. 5a ). However, the age models of the two cores differ, with regard to the onset of the deglacial B-P age decrease identified at ~18.8 cal. ka BP in core SO161-SL22. In fact, without information on potential changes in R surf , De Pol-Holz et al . [11] assumed a constant R surf of 400 years at site SO161-SL22 to establish the age model of the core. As shown above, the largest and longest period of the low B-P age difference in our record (between ca. 17 and 14 cal. ka BP) is associated with the highest observed R surf in the SEP during the last deglaciation, emphasizing the mixing of upper intermediate and surface waters with a 14 C-depleted deep-water mass. On the basis of these observations, the existence of a B-P age phase shift between both records appears questionable. Today, the SO161-SL22 site is under the influence of the surficial Peru–Chile current originating from the northern branch of the ACC. Thus, surface waters at MD07-3088 and SO161-SL22 sites should have undergone similar R surf changes. 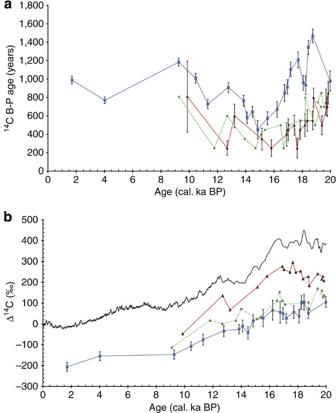Figure 5: South-Eastern Pacific waters14C activity. (a) Comparison between benthic–planktic radiocarbon age difference in core MD07-3088 (14C B-P age; this study; blue squares) and core SO161-SL122 (red triangles11) and recalculated14C B-P age in core SO161-SL122 using the variableRsurffrom this study (green circles). The error bars represent combined 1σ error in the14C dates. (b) Comparison of the atmospheric14C activity (Δ14C) from IntCal09 (black line) with oceanic14C activity (Δ14C) obtained from benthic foraminifera from core MD07-3088 (this study; blue squares), benthic foraminifera Δ14C from intermediate waters off Chile from core SO161-SL122 after De Pol-Holzet al.11(red triangles) and recalculated using the variableRsurffrom this study (green circles). Figure 5: South-Eastern Pacific waters 14 C activity. ( a ) Comparison between benthic–planktic radiocarbon age difference in core MD07-3088 ( 14 C B-P age; this study; blue squares) and core SO161-SL122 (red triangles [11] ) and recalculated 14 C B-P age in core SO161-SL122 using the variable R surf from this study (green circles). The error bars represent combined 1σ error in the 14 C dates. ( b ) Comparison of the atmospheric 14 C activity (Δ 14 C) from IntCal09 (black line) with oceanic 14 C activity (Δ 14 C) obtained from benthic foraminifera from core MD07-3088 (this study; blue squares), benthic foraminifera Δ 14 C from intermediate waters off Chile from core SO161-SL122 after De Pol-Holz et al . [11] (red triangles) and recalculated using the variable R surf from this study (green circles). Full size image By using a constant R surf age of 400 years in their age model, De Pol-Holz et al . [11] reconstructed an age-corrected AAIW Δ 14 C record displaying no significant depletion of the AAIW Δ 14 C values and suggesting no mixing with any hypothetical 14 C-depleted deep-ocean reservoir during the Heinrich 1 and/or the Younger Dryas periods ( Fig. 5b (ref. 11 )). In contrast, the reconstructed Δ 14 C values (at the lower boundary with AAIW) in the MD07-3088 record show a significant aging of these waters in the SEP at the onset of the deglaciation, which lasted until 16.7 cal. ka BP ( Fig. 5b ). In order to shed light on this point, we recalculated the Δ 14 C record from the northern Chile margin core SO161-SL22, using the R surf changes determined for MD07-3088. The derived ventilation ages are about twice as old as the original ones, revealing the degree to which unaccounted R surf variability may affect Δ 14 C calculations. This finding reveals an ageing of AAIW during the first deglacial warming (17.5–14.5 cal. ka BP) that is consistent with a reduction in the AAIW oxygen concentration at ocean drilling program (ODP) sites 1,233, 1,234 and 1,235 located at 41 °S and 36 °S, respectively ( Fig. 1 ; (ref. 14 )). The large difference between the ventilation age variations of AAIW calculated assuming a constant R surf [11] , and that calculated using the variable R surf derived here, demonstrates the importance of precisely determining R surf for the proper interpretation of marine Δ 14 C records. We therefore suggest that accurately mapping the spatial and temporal variability of R surf during the deglaciation should be a top priority for palaeoclimate studies. Study site Calypso core MD07-3088 was collected during the IMAGES PACHIDERME (MD 159) expedition by the French R/V Marion Dufresne in the SEP (46°04 S; 075°41 W; 1536, m; 18.9 m length; Fig. 1 ). Coring at this site recovered a fairly uniform succession of olive black to greyish olive diatom and silt-bearing clay for the upper 6 m. For the remaining 12.9 m, the sediment is dominated by greyish olive to grey silty clay with intercalations of silty/sandy layers. In this study, the first 17 m of the core are presented. The core location is within the ACC latitude belt under the direct influence of the northward Ekman transport of SSW ( Fig. 1a,b (ref. 16 )). Today, the study site is bathed by the upper layers of the nutrient-rich, oxygen-poor Pacific Central Waters at the boundary with the northward-flowing oxygen-rich AAIW. Stable isotopes Stable oxygen and carbon isotope ratios (δ 18 O, δ 13 C), expressed in ‰ versus VPDB (Vienna Pee Dee Belemnite standard) were obtained for the planktic foraminifera G. bulloides sampled every 5 cm. In addition, δ 13 C measurements were performed on the benthic foraminifera Cibicides wuellestorfii with a sampling resolution along the core every 10 cm. Six to ten shells were picked within the 250 to 315 μm size ranges for the planktonic analysis, one to four shells for the benthic analysis. Prior to isotopic analyses, the samples were cleaned in methanol using an ultrasonic bath for a few seconds then heated under vacuum at 380 °C for 45 min. Analyses were performed at Laboratoire des Sciences du Climat et de l'Environnement on Finnigan Delta+ and GV Isoprime mass spectrometers. VPDB is defined with respect to the NBS19 calcite standard [42] . The mean external reproducibility (1σ) of carbonate standards is ±0.06‰ for δ 18 O and±0.04‰ for δ 13 C; measured NBS18 is –23.2±0.2‰ VPDB for δ 18 O and −5.0±0.1‰VPDB for δ 13 C. The reproducibility for C. wuellestorfii and G. bulloides are 0.04 and 0.21‰ for δ 18 O and 0.06 and 0.23‰ for δ 13 C, respectively. The poor reproducibility for G. bulloides is because of the low number of specimens analysed, which prevent smoothing of the seasonal variation of the G. bulloides isotopic signal. However, the three-point average smoothed curve presented is closer to the annual mean signal. Sea surface temperatures Summer SSTs were determined using planktic foraminifera assemblages. Each sieved sample (>150 μm fraction) was split into 300–1,000 individuals for identification and counting. The SSTs were calculated using the Modern Analogue Technique [43] , a SO database [44] and the PaleoAnalogs software [45] . This method directly measures the difference between the faunal composition of a fossil sample and a modern database, and it identifies, for each fossil assemblage, the best modern analogues. Reliability of SSTs is estimated using a square chord distance test (dissimilarity coefficient) that represents the mean degree of similarity between the sample and the best 4–20 modern analogues. The calculated mean standard deviation of SST estimates observed in core MD07-3088 is ~1.5 °C during the last 20 ka. Geochemistry Marine ash layers were identified by the relative abundance of glass shards in core MD07-3088 as previously described [30] . Counting of glass shards from 210 samples was previously conducted on the detrital fraction every 10 cm along the core, with a resolution of 5 cm between 600 and 900 cm because of the occurrence of several eruptions closely spaced in time. Additional counts at higher resolution (every 1 cm) in core MD07-3088 between 275 and 285 cm permitted the identification of a new tephra layer at 278–279 cm ( Supplementary Fig. S2 ). Major-element analyses of individual glass shards were performed on CAMECA-SX 100 Electron Microprobe (EPMA-CAMPARIS) at the University Pierre et Marie Curie (UPCM, Paris VI). Radiocarbon dates 14 C dating was performed at UMS-ARTEMIS (Pelletron 3MV) AMS (CNRS-CEA Saclay, France) and at Keck Carbon Cycle Accelerator Mass Spectrometer facilities, University of California, Irvine. AMS 14 C measurements were performed on handpicked monospecific planktic and mixed benthic foraminifera in the size fraction >150 μm. Twenty-four dates were obtained for monospecific planktic foraminifera G. bulloides and 22 were obtained for mixed benthic foraminifera. AMS 14 C results are provided in Supplementary Tables S1,S2 . The age model for the core was derived from the calibrated planktic ages by applying a variable R surf correction (this study) and using the calibration program OxCal [25] at the 95% confidence level (2σ) based on IntCal09 (ref. 26 ) and IntCal04 (ref. 27 ). As this core has a very high sedimentation rate (~60 to 260 cm ka −1 ), bioturbation effects should be minimal. Finally, to compare the B-P foraminifera 14 C age of our core with the atmospheric 14 C history, we derived estimates of deep SEP Δ 14 C by using the following equation [46] : where 8,033 and 8,266 are the Libby and the true mean lives of 14 C, respectively. These values together with their 1σ uncertainties are listed in Supplementary Table S2 . Radiocarbon model simulation To examine the influence of the changing atmospheric Δ 14 C concentrations on the B-P ages at the location of core MD07-3088, we simulated the oceanic Δ 14 C over the last 26 ka in a global ocean circulation model. For this simulation, we used a data-constrained circulation model [47] , which has been fitted to modern hydrographic and tracer data. The model resolution is 2° in the horizontal with 24 unevenly spaced vertical levels. One of the model constraints is the pre-bomb radiocarbon concentration from the Global Ocean Data Analysis Project compilation [24] . The root mean squared model-data misfit for pre-bomb radiocarbon concentrations is 7.4%, and the relative error is 0.7 (a value <1 indicates that the model-data misfit is within the estimated uncertainty of the observations). We simulate Δ 14 C over the deglaciation following the methodology of De Vries and Primeau [48] . We define the tracer R =(Δ 14 C/1,000)+1, which is treated as a passive tracer that decays with an e-folding decay timescale of 8,266 years. Biological sources and sinks of R are neglected because their influence is small [49] . The only source of R in the ocean is because of gas exchange at the air–sea interface, where the flux of R is proportional to the atmospheric concentration R atm , Following De Vries and Primeau [48] , the piston velocity k is assumed to be proportional to the CO 2 piston velocity K w , where s is the solubility of CO 2 in seawater, p CO 2 is the partial pressure of atmospheric CO 2 and DIC is the mean surface dissolved inorganic carbon concentration. We use the CO 2 piston velocity from the Ocean Carbon Cycle Model Intercomparison Project Phase 2 protocol [50] , which is reduced by a factor of 20% to account for recent estimates [51] . Atmospheric p CO 2 is prescribed to follow the reconstructed history from the EDC and Vostok ice cores [52] . DIC is assumed to change by 1% for every 10% change in atmospheric p CO 2 , consistent with the average surface ocean buffer factor of ~10 (ref. 53 ). Reference values for the pre-industrial period are p CO 2 =280 μ atm and DIC=2 mmol m −3 (ref. 50 ). The solubility s is derived from modern temperature and salinity using the equation of Weiss [54] . Temporal variability in s is ignored because deglacial temperature and salinity records are sparse, and changes in s are likely to be smaller than the changes in p CO 2 . We perform two simulations; one in which the atmospheric history R atm is taken from the IntCal09 reconstruction [26] , and one in which we use R atm from the IntCal04 reconstruction [27] . We then calculate the B-P age from the modelled surface and deep-ocean Δ 14 C at the location of core MD07-3088. This B-P age record is the one that would be expected because of the observed changes in atmospheric Δ 14 C, if there were no changes in the ocean circulation. The difference then between the reconstructed B-P ages and the modelled B-P ages are due entirely to changes in circulation, having removed the influence of changing atmospheric Δ 14 C. Radiocarbon and δ 13 C as oceanographic tracers The δ 13 C of DIC and 14 C are both tracers of water masses. They are used together here as their distribution is not primarily controlled by the same factors. The δ 13 C distribution is controlled by the action of biology, which preferentially strips 12 C out of surface waters by ocean circulation that brings nutrients back into surface waters and by the exchange of CO 2 between the atmosphere and the ocean. The impact of air–sea exchange on the δ 13 C distribution depends on the rate of exchange and on the temperature of surface waters [55] . Biological and temperature fractionation effects are, however, negligible for the 14 C distribution, as they have very little effect compared with radioactive decay [49] , which lends a strong vertical gradient to the 14 C age distribution. The common mechanism that can affect vertical distributions of both Δδ 13 C and B-P 14 C age is oceanic vertical mixing: changes in the vertical gradient of Δδ 13 C and B-P 14 C age that are relatively rapid, synchronous and in the same direction (such as those observed during the upwelling periods highlighted in Fig. 3 ) are therefore most likely caused by changes in vertical mixing rates. How to cite this article: Siani, G. et al . Carbon isotope records reveal precise timing of enhanced Southern Ocean upwelling during the last deglaciation. Nat. Commun. 4:2758 doi: 10.1038/ncomms3758 (2013).